Discovery of a black smoker vent field and vent fauna at the Arctic Mid-Ocean Ridge The Arctic Mid-Ocean Ridge (AMOR) represents one of the most slow-spreading ridge systems on Earth. Previous attempts to locate hydrothermal vent fields and unravel the nature of venting, as well as the provenance of vent fauna at this northern and insular termination of the global ridge system, have been unsuccessful. Here, we report the first discovery of a black smoker vent field at the AMOR. The field is located on the crest of an axial volcanic ridge (AVR) and is associated with an unusually large hydrothermal deposit, which documents that extensive venting and long-lived hydrothermal systems exist at ultraslow-spreading ridges, despite their strongly reduced volcanic activity. The vent field hosts a distinct vent fauna that differs from the fauna to the south along the Mid-Atlantic Ridge. The novel vent fauna seems to have developed by local specialization and by migration of fauna from cold seeps and the Pacific. The discovery of the Trans-Atlantic Geotraverse (TAG) hydrothermal field on the Mid-Atlantic Ridge in 1985 [1] demonstrated that hydrothermal activity is not only restricted to ridges spreading at fast rates, but also occurs along parts of the global ridge system that are spreading at a slow rate (20–55 mm per year). At spreading rates below 20 mm per year, volcanic activity decreases to a level where the crust becomes thinner than normal and may even disappear—resulting in the upper mantle becoming exposed at the seafloor [2] , [3] . The magmatic heat budget at these ultraslow-spreading ridges is one order of magnitude below that at fast-spreading ridges [4] , and the extent that hydrothermal activity could be sustained at such ridges has been questioned. However, oceanographic surveys along parts of the South-west Indian Ridge and the Gakkel Ridge have shown that venting is more common than expected [5] , [6] , [7] . Further advances in our understanding of venting at ultraslow-spreading rates have been awaiting the discovery of specific venting sites and the sampling of fluids being released there. Chemoautotrophic primary production at submarine hot springs supports endemic vent fauna. The fauna at Pacific vent sites is distinct from that at Atlantic sites, and the discovery of a vent field at the East Indian Ridge revealed a mixed Atlantic and Pacific provenance [8] . This has been proposed to support the hypothesis of an along-ridge migration using active vent sites as stepping stones [9] , [10] , [11] . In the Atlantic, Iceland forms a barrier for northward along-ridge migration. Until now, four vent sites have been studied in the north of Iceland [12] , but these are all dominated by local bathyal species [13] . However, these vent sites are located at the southern part of the AMOR, which is influenced by the Icelandic hot spot, and therefore they are unusually shallow. As local bathyal species are known to replace vent endemic fauna at shallow water depths [14] , exploration of the deeper parts of the AMOR to the north was necessary to obtain conclusive information about the nature of vent fauna within the isolated Arctic Ocean. Here, we report the discovery of a black smoker vent field located at the AMOR. The field is associated with a large hydrothermal deposit and it hosts distinct fauna, which differs from that of the Mid-Atlantic Ridge. Geology of the Loki's Castle vent field In July 2008, we discovered a deep vent field 'Loki's Castle' on the AMOR at 73°30′N and 8°E ( Fig. 1 ), and revisited it in 2009 and 2010 for additional sampling. The vent field is located where the Mohns Ridge passes into the Knipovich Ridge through a sharp northward bend in the direction of the spreading axis. The venting occurs near the summit of an AVR that is around 30 km long, and the vent field is here associated with a 50–100-m deep rift that runs along the crest of the volcano ( Fig. 2 ). The field is composed of four active black smoker chimneys, up to 13 m tall, at the top of a mound of hydrothermal sulphide deposits. Venting of 310–320°C black smoker fluids occurs at two sites that are around 150 m apart. These venting areas seem to be located above two north-east-striking, semi-parallel normal faults that define the north-western margin of the rift. Two 20–30-m high sulphide mounds have developed around the venting areas. The mounds are each 150–200 m across at the base where they coalesce into a large composite mound. This is comparable in size to the TAG-mound, which is one of the largest hydrothermal mounds known to date in the deep ocean [15] . The main sulphide assemblage in chimneys consists of sphalerite, pyrite and pyrrhotite, with minor amounts of chalcopyrite. Some sulphide-poor samples are mostly composed of anhydrite, gypsum and talc. A gravity core taken from the mound sampled more Cu-rich hydrothermal deposits 0.5 m subsurface, indicating that higher temperature venting had occurred in the past. An area with low-temperature venting was located at the eastern flank of the mound. There, a dense field of small (<1 m) chimneys composed primarily of barite is associated with bacterial mats and a rich vent fauna. Clear, shimmering ∼ 20°C fluids are locally seen to emanate from this low-temperature field. 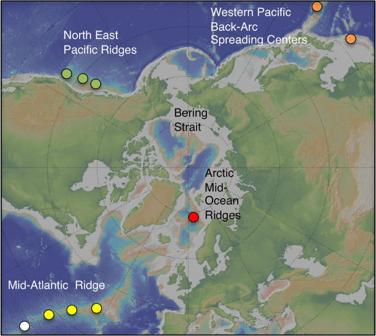Figure 1: Location of the Loki's Castle Vent field. A polar projection map showing the Arctic Mid-Ocean Ridge north of Iceland and the location of the Loki's Castle vent field (red dot). The map also shows the locations of the vent fields within the Atlantic and the Pacific ocean hosting vent endemic fauna belonging to different biogeographic provinces: white, Mid-Atlantic Ridge; yellow, Azores; orange, Western Pacific; green, North-East Pacific (biogeographic provinces from ref.11). Figure 1: Location of the Loki's Castle Vent field. A polar projection map showing the Arctic Mid-Ocean Ridge north of Iceland and the location of the Loki's Castle vent field (red dot). The map also shows the locations of the vent fields within the Atlantic and the Pacific ocean hosting vent endemic fauna belonging to different biogeographic provinces: white, Mid-Atlantic Ridge; yellow, Azores; orange, Western Pacific; green, North-East Pacific (biogeographic provinces from ref. 11 ). 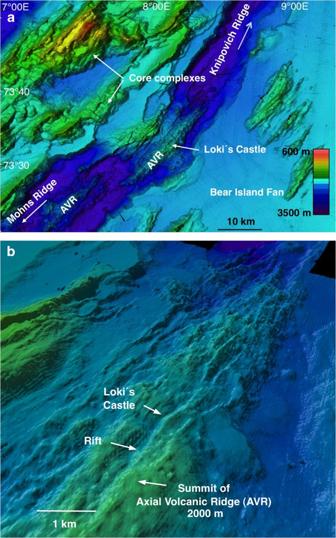Figure 2: Geology of the Eastern Mohns Ridge. (a) Map showing: (1) the 30-km-long AVR hosting the vent field; (2) core complexes at the western flank of the ridge; and (3) the eastern flank that is buried by the distal parts of the Bear Island sedimentary fan, which developed during repeated Arctic glaciations during the last 3 million years. (b) Bathymetry of the AVR and surrounding terrain viewed obliquely from the south. The map shows that the vent field is located next to a rift that runs along the crest of the ridge, where normal faults appears to represent the main channel way for the hydrothermal fluids. Full size image Figure 2: Geology of the Eastern Mohns Ridge. ( a ) Map showing: (1) the 30-km-long AVR hosting the vent field; (2) core complexes at the western flank of the ridge; and (3) the eastern flank that is buried by the distal parts of the Bear Island sedimentary fan, which developed during repeated Arctic glaciations during the last 3 million years. ( b ) Bathymetry of the AVR and surrounding terrain viewed obliquely from the south. The map shows that the vent field is located next to a rift that runs along the crest of the ridge, where normal faults appears to represent the main channel way for the hydrothermal fluids. Full size image Vent fluid compositions The Loki's Castle high-temperature vent fluids ( Table 1 ) have high volatile concentrations (CO 2 =26.0, CH 4 =15.5, H 2 =5.5; all in mmol kg −1 ). The CH 4 values are among the highest reported from a volcanic-hosted field. The high CH 4 and H 2 values could indicate interaction with ultramafic rocks [16] , [17] . However, the ultramafic systems studied to date exhibit higher concentrations of H 2 (up to 15–16 mmol kg −1 ) and lower CH 4 /H 2 ratios [16] , [17] , [18] . The Loki's Castle fluids are further characterized by a pH of 5.5, end-member (EM) hydrogen sulphide (H 2 S) content up to 4.7 mmol kg −1 and very high ammonium (NH 4+ ) concentrations (6.1 mmol kg −1 ). The high CH 4 values together with the elevated NH 4+ concentrations point to a sedimentary influence. Significant sediment accumulations are not present at the volcanic ridge hosting the field, but the distal parts of a sedimentary fan are present 5 km to the south-east ( Fig. 2 ). Sediments at depth below the volcano seem to be the most likely source of the anomalous volatile contents. Table 1 EM compositions of hydrothermal fluids. Full size table Vent fauna Loki's Castle harbours a rich, locally adapted and specialized, deep-water vent fauna. Dense fields of siboglinid tube worms ( Sclerolinum contortum ) on the sulphide mound ( Fig. 3a,b ) are among the organisms that dominate in terms of abundance and biomass. These are normally found on cold seeps and are common at the nearby Haakon Mosby Mud Volcano and the Nyegga cold seeps. Molecular markers support the morphological identification, and the hot vent and cold seep individuals differ by <1% in the cytochrome c oxidase subunit I gene sequences (the Folmer fragment) [19] . A recent molecular analysis of S. contortum from the Håkon Mosby Mud Volcano yielded only evidence for sulphur-oxidizing symbionts [20] . 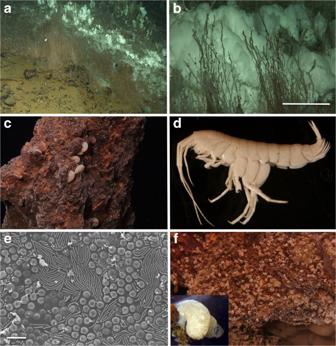Figure 3: Characteristic invertebrates at the Loki's Castle vent field. (a) Siboglinid tubeworms (S. contortum) associated with low-temperature diffuse venting at the flank of the hydrothermal mound. White microbial mats and small barite chimneys in the back. (b) Close-up of the siboglinid tube worms in front of white microbial mats. Note the dense populations of small gastropods (P. griegiandSkeneasp.) on the tubes. The scale bar is 5 cm. (c) Amphipods (Melitidae sp. nov.) on a chimney wall. (d) Close-up of a∼1.5 cm juvenile Melitid amphipod. (e) Scanning electron microscopic image of chemoautotrophic gill symbionts from the Melitid amphipod (the scale bar is 3 μm). Based on 16S rDNA clone libraries, the two most abundant sequences are affiliated with a gamma proteobacterium, known as a sulphur oxidizer in the bivalveAnodontia fragilis, and sequences with 98% similarity to an uncultured Methylococcaceae known as a methanotrophic ectosymbiont on the vent crabShinkaia crosnieri. (f) Small gastropods (P. griegi) populating a chimney wall, with an individual shown as an inset picture (∼3 mm across). Figure 3: Characteristic invertebrates at the Loki's Castle vent field. ( a ) Siboglinid tubeworms ( S. contortum ) associated with low-temperature diffuse venting at the flank of the hydrothermal mound. White microbial mats and small barite chimneys in the back. ( b ) Close-up of the siboglinid tube worms in front of white microbial mats. Note the dense populations of small gastropods ( P. griegi and Skenea sp.) on the tubes. The scale bar is 5 cm. ( c ) Amphipods (Melitidae sp. nov.) on a chimney wall. ( d ) Close-up of a ∼ 1.5 cm juvenile Melitid amphipod. ( e ) Scanning electron microscopic image of chemoautotrophic gill symbionts from the Melitid amphipod (the scale bar is 3 μm). Based on 16S rDNA clone libraries, the two most abundant sequences are affiliated with a gamma proteobacterium, known as a sulphur oxidizer in the bivalve Anodontia fragilis , and sequences with 98% similarity to an uncultured Methylococcaceae known as a methanotrophic ectosymbiont on the vent crab Shinkaia crosnieri . ( f ) Small gastropods ( P. griegi ) populating a chimney wall, with an individual shown as an inset picture ( ∼ 3 mm across). Full size image A putative new species of amphipod, which requires further verification, within the Melitidae group is a characteristic member of this community ( Fig. 3c,d ). These amphipods are found in crevices on the chimneys and in the tube worm fields. They have two main populations of chemoautotrophic gill symbionts ( Fig. 3e ). A δ 15 N value of −5.9‰ shows a trophic relationship to microbial populations. A δ 34 S isotope signature of +11.9‰ is consistent with this, whereas the carbon isotope ratio is less diagnostic (δ 13 C=−23‰). The new amphipod species seems to represent a local Arctic adaptation to a trophic niche that in the Atlantic Ocean is filled by vent shrimps. The chimney walls are also densely populated by small grazing gastropods Pseudosetia griegi ( Fig. 3f ) and Skenea spp. P. griegi is also known from the Jan Mayen vent fields and the Nyegga cold seeps [13] . Thick crusts of tube-dwelling polychaetes ( Nicomache sp nov.) are found at diffuse venting sites at the base of some chimneys and at the sulphide mound. Similarly, vent-adapted species of Nicomache are known from the Eastern Pacific as far north as the Explorer Ridge [21] . The Stauromedusae Lucernaria bathyphila was found surrounding outlets of moderately warm fluids. Only one other species of this group ( Lucernaria janetae ) is known from such depths. This was associated with a black smoker vent field at the East-Pacific Rise [22] . The sheer size of the mound at Loki's Castle documents extensive venting and shows that ultraslow-spreading ridges may host unusually large hydrothermal deposits despite their reduced magmatic heat budget. The longevity of vent fields depends on the size of the heat source and the stability of the conduit. The importance of long-lived detachment faults for hydrothermal activity at slow-spreading ridges has recently been recognized [23] , [24] , [25] . The Loki's Castle field shows that long-lived conduits may also form directly at the AVRs ( Fig. 4a ), probably as a result of the slow plate divergence and the reduced volcanic activity at ultraslow-spreading rates. 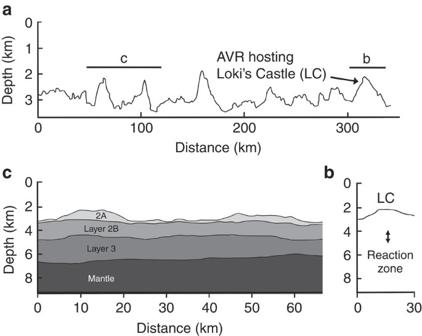Figure 4: Depth of reaction zone and lithospheric structure. (a) Along-axis profile of the central and eastern part of the Mohns Ridge showing the variations in water depth. The profile shows the 30-km-long and 800-m-high AVR hosting the Loki's Castle vent field and the distribution of similar AVRs to the south-west along the ridge. The lines marked b and c show the locations of the along-axis profiles shown inbandc. (b) Profile of the water depth along the AVR hosting Loki's Castle, and the subsurface depth of the reaction zone, as estimated by EM vent fluid composition using a Si-Cl geothermobarometer27. The estimated depth of the reaction zone corresponds to the seismic layer 2–3 transition as seen further west at the Mohns Ridge (c). The depth of the reaction zone combined with the crustal thickness suggests that as much as 50% of the crust is convectively cooled by hydrothermal circulation. (c) Seismic structure across two of the AVRs shown ina(marked c) that document the unusually thin ocean crust (∼4 km) and the boundary between the different oceanic layers within the crust (data from ref.28). Figure 4: Depth of reaction zone and lithospheric structure. ( a ) Along-axis profile of the central and eastern part of the Mohns Ridge showing the variations in water depth. The profile shows the 30-km-long and 800-m-high AVR hosting the Loki's Castle vent field and the distribution of similar AVRs to the south-west along the ridge. The lines marked b and c show the locations of the along-axis profiles shown in b and c . ( b ) Profile of the water depth along the AVR hosting Loki's Castle, and the subsurface depth of the reaction zone, as estimated by EM vent fluid composition using a Si-Cl geothermobarometer [27] . The estimated depth of the reaction zone corresponds to the seismic layer 2–3 transition as seen further west at the Mohns Ridge ( c ). The depth of the reaction zone combined with the crustal thickness suggests that as much as 50% of the crust is convectively cooled by hydrothermal circulation. ( c ) Seismic structure across two of the AVRs shown in a (marked c) that document the unusually thin ocean crust ( ∼ 4 km) and the boundary between the different oceanic layers within the crust (data from ref. 28 ). Full size image Vent fields are less frequent at ultraslow-spreading ridges than at ridges spreading at faster rates. This is related to the magmatic heat being strongly reduced as a result of the lower spreading rates and thinner crust. However, relative to the magmatic heat available, the frequency of hydrothermal vent sites seems to be 2–3 times higher at ultraslow-spreading ridges than at ridges spreading at faster rates [4] . The reason for this is unclear, but tapping of deeper heat sources within the lower crust or upper mantle has been proposed [4] . The Loki's Castle fluids reach 317°C, with an EM SiO 2 content of up to 16 mmol kg −1 . EM chlorinity is around 85% of seawater suggesting that the fluids have phase separated at depth. The SiO 2 and chlorinity contents of vent fluids are pressure and temperature sensitive [26] , [27] . The fluid compositions indicate that the rock-water reactions occur around 2 km below the seafloor ( Fig. 4b ). This is comparable to the depth of the reaction zones at ridges spreading at a much faster rate [27] . The crustal thickness is estimated to be 4±0.5 km at the central Mohns Ridge [28] ( Fig. 4c ). This is 2–3 km less than the average thickness of oceanic crust. Therefore, the depth of the reaction zone is comparable to fast-spreading ridges; however, the fraction of crust cooled convectively by hydrothermal circulation is two times that of vent fields at ridges with normal crustal thickness. The chemoautotrophic primary production at Loki's Castle supports a vent fauna that is different from that found further south in the Atlantic, where shrimps, large bivalves and crabs are abundant [29] . This lack of typical Atlantic vent fauna indicates either an unfavourable environment or migrational barriers. The ambient water temperature at this Arctic site (−0.7°C) represents one obvious environmental difference. Iceland defines a land barrier for along-axis dispersal of fauna, and a southerly flow of deep water from the Arctic represents an additional barrier for deep-water migration northwards. The Arctic Ocean is relatively isolated from the rest of the world's oceans and a high degree of endemism in the deep-water fauna is well documented [30] , [31] . This endemism clearly extends to the hot-vent environment. The presence of siboglinid tube worms at Loki's Castle documents interactions between the hot vents and cold-seeps. Several factors may favour such interactions in the Arctic: (1) the general proximity of the ridge system to the continental margins; (2) the unusually high methane concentrations in vent fluids, as documented at Loki's Castle, resulting from interaction between hydrothermal fluids and glacimarine sedimentary deposits; and (3) reduced or arrested methane release from the continental shelf during periods of glaciations [32] —rendering the hot vents as safe havens for chemosynthetic organisms during Arctic glaciations. Some species found at Loki's Castle are closely related to species known from vent sites in the Northern Pacific (for example, the polychaetes Nicomache sp nov. and Amphisamytha sp). Seawater enters the Arctic Ocean either as the North-Atlantic current that bring warm surface water into the Arctic from the south, or as a flow of colder water through the Bering Strait from the Pacific Ocean ( Fig. 1 ). The Bering Strait first opened at 4.8–5.5 Ma, and the abrupt appearance of North-Pacific molluscs in the North Atlantic occurred at 3.6 Ma [33] . Our present data therefore indicate that the fauna composition is a result of locally adapted species and of migration from cold seep environments in combination with recent migration of vent fauna into the Arctic Ocean from the Pacific Ocean. The discovery of this Arctic vent field provides a new opportunity to advance our understanding of the migration of vent fauna and interactions between different chemosynthetic deep-sea environments. The new Arctic vent field also provides the first insight into hydrothermal systems at ultraslow-spreading ridges, which make up 20% of the global ridge system. Bathymetry Bathymetry was acquired by R/V G.O. Sars using a Kongsberg Simrad EM300 multibeam echo sounder system. The data processing was done with Kongsberg Simrad Neptune software, the data were gridded to 30 m cell sizes and were displayed using the Fledermaus software package. Water column analyses Potential venting areas were selected based on the bathymetry, and the water column above these areas were searched for signs of venting using a Seabird conductivity/temperature/depth profiler that was equipped with a particle sensor (C Star transmissometer), and an Eh-sensor that was kindly provided by Koichi Nakamura (Geol. Surv. of Japan, Agency of Ind. Sci. and Technol). Plume samples for methane and hydrogen were analysed by a headspace technique in which 100 ml of sample and 40 ml of helium were combined in a 140 ml syringe. The sample was vigorously shaken and allowed to equilibrate until the sample reached room temperature. The analysis was done by gas chromatography using a pulsed discharge detector for hydrogen and a flame ionization detector for methane. Remotely operated vehicle (ROV) operations and sampling The vent field was located and sampled using a Bathysaurus XL remotely operated vehicle (ROV) provided by Argus Remote Systems. Video was acquired using a high-definition camera, from which the still photos were captured. Fluid samples were collected using 250 and 1,000-ml titanium syringe samplers. Fluids for gas analyses were collected in pre-evacuated titanium gas tight samplers. The vent fauna was sampled by a suction sampler and with a hydraulically operated box sampler. High-temperature vent fluid analyses H 2 S and NH 4+ as well as pH were measured onboard. The subsamples analysed for H 2 S were drawn in a vial and fixed immediately with reagents for the photometric methylene blue method. NH 4+ analyses were done using the photometric indophenol method. Chloride was analysed onshore by ion chromatography, and magnesium and silica were quantified by inductively coupled plasma optical emission spectrometry. On recovery, the gas tight samplers were connected to a shipboard vacuum line and the gases were extracted, dried and sealed in break-seal glass tubes. Several cuts of each sample were taken and CO 2 , CH 4 and H 2 contents were analysed in shore-based laboratories. The Mg contents of the different samples provided information on the relative amount of hydrothermal fluid and seawater in the samples taken. The Mg value of the sample was then used to calculate the vent fluid composition (called EM vent fluid composition), shown in Table 1 . DNA and stable isotope analyses The C, N and S isotope compositions of vent fauna taxa were analysed at Institute for Energy Technology (IFE), Norway. Approximately 1 mg of material was used for the C and N analyses and 2 mg for the S analyses. The isotopic measurements were done with a Nu Instrument Horizon, isotope ratio mass spectrometer, and the results were corrected against international standards IAEA-N-1 and IAEA-N-2 (δ 15 N), USGS-24 (δ 13 C), and IAEA-S1 and IAEA-S2 for δ 34 S analyses. DNA was extracted using the FastDNA SPIN Kit for Soil following the protocols from the supplier. The Folmer primers were used to amplify a 550-bp region of cytochrome c oxidase subunit I. The 16SrDNA clone library of gill symbionts in the melitid amphipod was obtained using the primers B338f [34] and B1392r (modified from ref. 35 ) and the Strataclone PCR Cloning Kit from Strategene. Scanning electron microscopic micrographs of gill symbionts were prepared using a ZEIZZ Supra 55VP FE-SEM on critical point-dried and iridium-coated material. How to cite this article: Pedersen, R.B. et al . Discovery of a black smoker vent field and vent fauna at the Arctic Mid-Ocean Ridge. Nat. Commun. 1:126 doi: 10.1038/ncomms1124 (2010).